Top–down fabrication of sub-nanometre semiconducting nanoribbons derived from molybdenum disulfide sheets Developments in semiconductor technology are propelling the dimensions of devices down to 10 nm, but facing great challenges in manufacture at the sub-10 nm scale. Nanotechnology can fabricate nanoribbons from two-dimensional atomic crystals, such as graphene, with widths below the 10 nm threshold, but their geometries and properties have been hard to control at this scale. Here we find that robust ultrafine molybdenum-sulfide ribbons with a uniform width of 0.35 nm can be widely formed between holes created in a MoS 2 sheet under electron irradiation. In situ high-resolution transmission electron microscope characterization, combined with first-principles calculations, identifies the sub-1 nm ribbon as a Mo 5 S 4 crystal derived from MoS 2 , through a spontaneous phase transition. Further first-principles investigations show that the Mo 5 S 4 ribbon has a band gap of 0.77 eV, a Young’s modulus of 300GPa and can demonstrate 9% tensile strain before fracture. The results show a novel top–down route for controllable fabrication of functional building blocks for sub-nanometre electronics. Developments in micro-nanofabrication technologies, including optical lithography, electron beam lithography, focused ion beam technique, X-ray lithography and various etching and replication techniques, are essential for a variety of industry fields. These range from large-scale integrated circuits, optoelectronics and high-density magnetic storage to micro-electro-mechanical systems and nanotechnology. These top–down technologies have recently led the semiconductor industry into a 22-nm generation, but it remains a great challenge to controllably fabricate sub-10 nm structures. Thinning bulk material to single-atomic layers has led us into a two-dimensional (2D) crystal age [1] , [2] , [3] . To further narrow 2D crystals into functional nanoribbons is attracting our current attention and effort. The three main methods of unwrapping nanotubes [4] , [5] , cutting 2D sheets [6] , [7] and self-assembly of small molecules into ribbons [8] , have been used for fabrication of graphene or boron nitride nanoribbons, but it is still difficult to fabricate very narrow semiconducting nanoribbons with uniform geometry. The 2D transition metal dichalcogenides have been studied for decades for their electronic, optical and catalytic properties as well as specific mechanical properties [2] , [9] , [10] , [11] , [12] , but how to shape them into nanoribbons has hardly been studied [13] , [14] . Here, we find a novel approach to fabricate uniform and robust semiconducting molybdenum-sulfide ribbon with sub-nanometre width simply by in situ electron irradiation in a transmission electron microscope (TEM). It is shown that the sulphur atoms at the edge of a MoS 2 sheet are too fragile to withstand the electron beam irradiation, so that holes, once created, can rapidly spread towards each other and produce ribbons between them. When the ribbon width is narrowed to a critical size below 1 nm, phase transition into a distinctly robust Mo 5 S 4 structure occurs spontaneously before the holes can coalesce. This approach could be developed into a general controllable method for fabrication of sub-1 nm building blocks from transition metal dichalcogenide sheets for future functional devices. In situ fabrication of ultrafine molybdenum-sulfide ribbon The in situ electron irradiation experiment at room temperature started with a MoS 2 monolayer (S-Mo-S triple atom layers) prepared by micromechanical cleavage as identified by both optical ( Fig. 1a and Supplementary Fig. S1 ) and high-resolution TEM (HRTEM) characterization ( Fig. 1b ). Under the irradiation of electron beam, defects can be created in the thin 2D sheet once the beam energy exceeds the knock-on damage threshold of the sheet [15] . 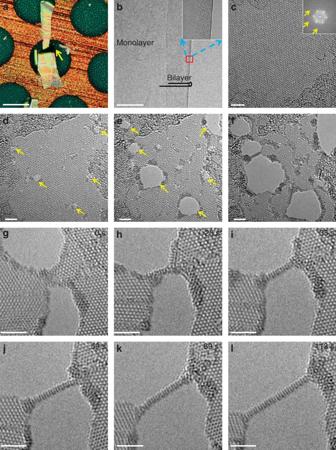Figure 1:In situfabrication of suspended molybdenum-sulfide sub-nanometre ribbons. (a) A few-layer MoS2flake on TEM grid. The thinnest region locates at the region labelled by arrow. Scale bar, 100 μm. (b) TEM images of the thinnest region. The thickness of the membrane can be determined by fringe counting at the edge. The straight edge verifies that the membrane is single layer. The folded and unfolded region can be further determined by contrast. Scale bar, 100 nm. (c) High-resolution TEM data obtained on the unfolded regions. The corresponding fast Fourier transformation (FFT) image is shown in the inset. (d) The initial MoS2membrane with small irradiation-induced vacancies as highlighted by the arrows. (e,f) Larger holes extended from the small vacancies upon 80 kV electron irradiation of another 108 and 261 s. (g–l) Time series of the formation and growth for a suspended sub-nanometre ribbon under 80 kV electron irradiation. In (c–l) scale bar, 2 nm. The energy for removing sulphur and molybdenum atoms in a perfect MoS 2 sheet are calculated by first-principles calculations to be 6.1 and 13.9 eV ( Table 1 ), respectively. Once a hole is created in the sheet, the energy for removing a sulphur atom from an armchair or zigzag edge is significantly reduced to 4.9 or 4.4 eV, respectively. As the maximum energy transferred from an 80 kV electron to a sulphur atom is about 6 eV ( Supplementary Fig. S2 ), which is between the thresholds of the edge and the interior sulphur vacancies of the MoS 2 sheet, we chose an acceleration voltage of 80 kV to achieve enough resolution, while maintaining the MoS 2 sheet in highly crystalline condition. The electron beam was firstly focused to 40 A cm −2 to induce initial defects and holes in the MoS 2 sheet. After 81 s irradiation, small vacancy aggregations formed as labelled by the arrows in Fig. 1d . As the edge of the defects was much weaker, all the defects spread rapidly in exposure to the irradiation. After another 103 s irradiation, the defects extended into holes with diameters of 3–6 nm as shown in Fig. 1e , with an average edge shrinking speed of about 0.02 nm s −1 . Along with the growth of holes, the connecting regions between them were narrowed into nanoribbons, showing a trend for coalescence. But just before the coalescence occurred, the thinnest connecting ribbon spontaneously turned into a fine ribbon with smooth edges and uniform width of 0.35 nm ( Fig. 1f ), which was robust to the dense electron irradiation ( Supplementary Fig. S3 for details). On the other hand, as the maximum transferred energy to Mo atoms (~2.0 eV) is much less than the threshold for removing Mo atoms, aggregation of molybdenum at the edges of holes, especially at the ends of the nanoribbons, can be found ( Fig. 2 ). Figure 1: In situ fabrication of suspended molybdenum-sulfide sub-nanometre ribbons. ( a ) A few-layer MoS 2 flake on TEM grid. The thinnest region locates at the region labelled by arrow. Scale bar, 100 μm. ( b ) TEM images of the thinnest region. The thickness of the membrane can be determined by fringe counting at the edge. The straight edge verifies that the membrane is single layer. The folded and unfolded region can be further determined by contrast. Scale bar, 100 nm. ( c ) High-resolution TEM data obtained on the unfolded regions. The corresponding fast Fourier transformation (FFT) image is shown in the inset. ( d ) The initial MoS 2 membrane with small irradiation-induced vacancies as highlighted by the arrows. ( e , f ) Larger holes extended from the small vacancies upon 80 kV electron irradiation of another 108 and 261 s. ( g – l ) Time series of the formation and growth for a suspended sub-nanometre ribbon under 80 kV electron irradiation. In ( c – l ) scale bar, 2 nm. Full size image Table 1 The non-relaxed formation energies of chalcogen and metal vacancies E f (eV). 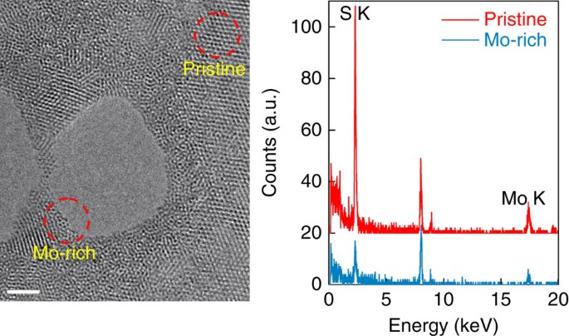Figure 2: Evidence for Mo-rich cluster at the edge of nanoribbon. The energy dispersive X-ray (EDX) spectrum indicates that S atoms are sputtered while Mo atoms aggregate. Scale bar, 2 nm. Full size table Figure 2: Evidence for Mo-rich cluster at the edge of nanoribbon. The energy dispersive X-ray (EDX) spectrum indicates that S atoms are sputtered while Mo atoms aggregate. Scale bar, 2 nm. Full size image To carefully investigate the surprising fine ribbon, we decreased the beam intensity to 10 A cm −2 . The typical formation and elongation process for a fine ribbon was recorded in Fig. 1g–l . The formed ribbon showed uniform width with identical atomic structures, in sharp contrast to the mother MoS 2 at its ends. Estimations from intensity profile curves suggested that the formed ribbon has a lattice distance of 0.44–0.46 nm in axial and 0.26–0.27 nm spacing between two palpable lattice sites in width ( Fig. 3a ). The lattice constants are distinctly different from those of any known molybdenum disulphide ribbon, indicating that a novel phase transition took place during the formation of the fine ribbon. In sharp contrast to the fragile MoS 2 ribbons, this sub-nanometre ribbon showed remarkable dynamic stability and were widely formed in our experiments on monolayer or few-layers MoS 2 samples ( Supplementary Fig. S4 ). 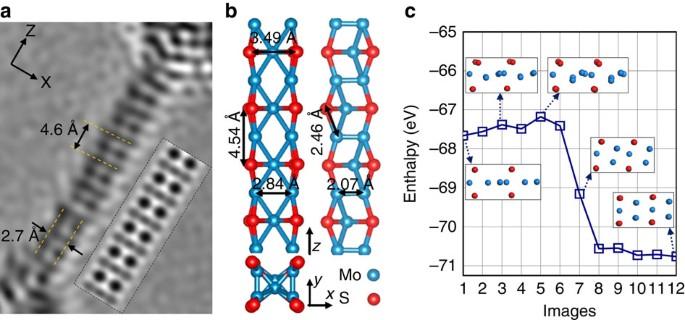Figure 3: Atomic structure and simulated formation process of the Mo5S4nanoribbon. (a) Comparison between the HRTEM micrograph and the simulated TEM micrograph (labelled by the dotted rectangle) of Mo5S4. To enhance the visibility of the ribbon structure, a low pass Fourier filter (7 nm−1) was applied to the HRTEM image. (b) Three view depictions of the Mo5S4ribbon. (c) Transition state simulation with 12 intermediate images for forming Mo5S4nanoribbon from a S-impoverished armchair ribbon. The enthalpy stands for the intermediate energy per primitive cell. Figure 3: Atomic structure and simulated formation process of the Mo 5 S 4 nanoribbon. ( a ) Comparison between the HRTEM micrograph and the simulated TEM micrograph (labelled by the dotted rectangle) of Mo 5 S 4 . To enhance the visibility of the ribbon structure, a low pass Fourier filter (7 nm −1 ) was applied to the HRTEM image. ( b ) Three view depictions of the Mo 5 S 4 ribbon. ( c ) Transition state simulation with 12 intermediate images for forming Mo 5 S 4 nanoribbon from a S-impoverished armchair ribbon. The enthalpy stands for the intermediate energy per primitive cell. Full size image Identification of crystal structure In what follows, we performed extensive structure search by first-principles calculations to determine the crystal structure of the irradiation-induced fine ribbon. As the fine ribbon consists of at most three lattice sites in width as indicated by the HRTEM intensity profile in Fig. 3a , we concentrated on ribbon structures with three or less columns of atoms at each cross section. Meanwhile, we presumed that the ratio of molybdenum to sulphur in this ribbon could vary from 2:1 to 1:0 because the fine ribbons were formed in a Mo-rich atmosphere ( Fig. 2 ). The optimized structures of the candidate ribbons and their lattice constants are summarized in Supplementary Fig. S5 and Supplementary Table S1 . It is found that only a Mo 5 S 4 ribbon with an axial constant of 0.45 nm and a separation of 0.28 nm between the two Mo atoms along the width direction ( Fig. 3b ) can exclusively match the experimentally estimated parameters of the observed fine ribbon. Moreover, the simulated HRTEM image based on the Mo 5 S 4 model is in good agreement with the experimental one, as compared in Fig. 3a . All the other searched structures differ far from the experimental results in either the lattice parameters or simulated TEM image. To shed light on the formation mechanism of the Mo 5 S 4 structure, transition state simulations from a MoS 2 ribbon to the Mo 5 S 4 ribbon were performed. When started from an armchair MoS 2 ribbon consisting of five dimer lines across width but with six sulphur atoms removed per unit cell ( Supplementary Fig. S6 ) in view of that the sulphur atoms can be easily knocked off from the ribbon edges, the phase transition into the targeted Mo 5 S 4 ribbon can be uniquely achieved via a rotation of two Mo–Mo dimers ( Fig. 3c ). Importantly, this phase transition occurs with a very low energy barrier of about 0.05 eV per atom, indicating that the initial sulphur-deficient armchair ribbon is likely to transform into the Mo 5 S 4 structure upon the irradiation. Furthermore, the formation energy for a sulphur vacancy in this sub-nanometre ribbon is calculated to be 6.8 eV, even over 11% higher than that of a perfect MoS 2 monolayer ( Table 1 ), justifying Mo 5 S 4 ’s robustness to the 80 kV electron irradiation. Mechanical and electronic properties of Mo 5 S 4 ribbon Under continuous 80 kV electron beam irradiation, the sub-nanometre Mo 5 S 4 ribbon can grow to tens of nanometres in length before breaking ( Supplementary Movie 1 ), indicating an excellent mechanical strength. Our first-principles simulations also predict that the ribbon has a respectable tensile strength up to 30 GPa and can be stretched for 9% before breaking without plastic deformation ( Fig. 4a ). Its Young’s modulus is calculated by fitting the linear elastic region of stress-strain curve to be about 300 GPa, close to that of pure MoS 2 sheets [16] . Further calculations on the Mo 5 S 4 ribbon with hybrid functional predict an indirect band gap with a desirable value of 0.77 eV ( Fig. 4b ). This gap value not only promises the optical adsorption into the infrared region but also can afford the logic operation of corresponding field-effect devices. Interestingly, the charge densities of valance band maximum and conduction band minimum orbitals exhibit a periodic fluctuation of two unit cells, which is due to the alternate vertical deviation of the interior Mo atoms from the center of the S rectangles ( Fig. 3b ) and indicates an origin of the band gap by Peierls distortion of 1D structure ( Supplementary Fig. S7 ). 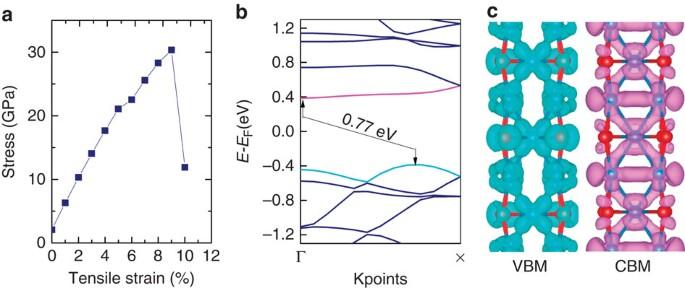Figure 4: Mechanical and electronic properties of the Mo5S4ribbon. (a) Strain–stress curve in a first-principles tensile simulation. (b) Electronic band structure of the Mo5S4nanoribbon. (c) Valance band maximum and conduction band minimum orbitals with an isosurface of 0.0015 e per Å3. Figure 4: Mechanical and electronic properties of the Mo 5 S 4 ribbon. ( a ) Strain–stress curve in a first-principles tensile simulation. ( b ) Electronic band structure of the Mo 5 S 4 nanoribbon. ( c ) Valance band maximum and conduction band minimum orbitals with an isosurface of 0.0015 e per Å [3] . Full size image As the transition metal dichalcogenides (MX 2 , TMDs) have similar structures and properties, similar sub-nanometre ribbons may be fabricated from them through the same mechanism by energy beam based irradiation or lithography technologies. To show this propensity, we conducted further first-principles calculations for the formation energies of chalcogen and metal vacancies in other 2D TMDs, such as WS 2 and MoSe 2 monolayers, the armchair and zigzag nanoribbons as well as similar M 5 X 4 sub-nanometre ribbons. It is found that, akin to the case of MoS 2 , the chalcogen atoms at the edge of armchair or zigzag ribbons are found to be the most fragile ones, while those in the M 5 X 4 ribbons remain robust. So the top–down method demonstrated by knocking a MoS 2 sheet into uniform robust sub-nanometre ribbons can likely be developed into a general methodology for controllable fabrication of many similar TMD ribbons. The formation energy differences presented also show the possibility to knock the TMDs into robust sub-nanometre ribbons by ion or other energy beams. 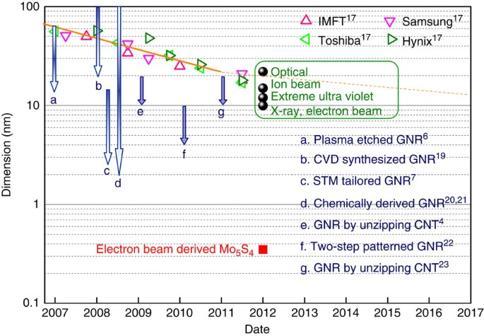Figure 5: Dimension distributions of nanostructures in semiconductor industry and nanotechnology. The triangles and solid circles stand for the reported dimension of flash 1/2 pitch17and lithography resolutions, respectively. The solid and dot lines are the time lines of flash industry18. Figure 5 shows the roadmap of semiconductor industry [17] , [18] and nanotechnology community to manufacture narrower functional nanostructures. The development in micro-nanofabrication technologies are propelling the dimension of flash down to 10 nm, but facing great challenges in manufacture at sub-10 nm scale. On the other hand, CVD grown [19] , STM tailored [7] and sonochemical derived [20] , [21] graphene nanoribbons can be ranged well into sub-10 nm, but the distributions of widths are quite scattered as shown by the arrows in Fig. 5 and the edges are rough when the ribbon width is down to 5 nm ( [22] , [23] ). Distinctively, the irradiation-derived robust sub-nanometre Mo 5 S 4 ribbon has a unique width, smooth edges and suitable band gap, which are vital to serve as building blocks for functional devices. Moreover, if the initial defects and holes in a MoS 2 layer can be induced in a controlled manner, it will be also possible to fabricate ordered array or networks of the sub-nanometre ribbons. Therefore, there are still a lot of attractive possibilities waiting for attempts along this route for a blueprint toward producing sub-nanometre electronics. Figure 5: Dimension distributions of nanostructures in semiconductor industry and nanotechnology. The triangles and solid circles stand for the reported dimension of flash 1/2 pitch [17] and lithography resolutions, respectively. The solid and dot lines are the time lines of flash industry [18] . Full size image Preparation and characterization of molybdenum disulphide monolayer The monolayer MoS 2 samples are exfoliated by micromechanical cleavage techniques from commercially available crystals of molybdenite (SPI Supplies Brand moly disulphide) and transferred to a TEM grid with support films of formvar and carbon using PMMA-based transfer method [24] . In order to remove the possible polymer residue, the samples are annealed at 200 °C in a mixture of hydrogen and argon before inserted into a TEM for further experiments. HRTEM was carried out using an image aberration-corrected TEM (FEI Titan 80-300 operating at 80 kV acceleration voltage), and a charge coupled device camera (2k × 2k, Gatan UltraScan 1000) is used for image recording with an exposure time of 1~2 s. Multislice image simulation [25] was performed with spherical aberration=1 μm, focus spread=2.16 nm, illumination semi-angle=0.5 mrad and defocus of 8 nm. Computational methods The first-principles calculations were performed within the framework of density functional theory as implemented in the VASP code [26] , [27] . We used doubled primitive cell of ribbons in structure optimizations for possible reconstructions and the systems were fully relaxed without any constraint. The projector augmented wave method [28] , [29] for the core region and the generalized gradient approximation of the PBE functional for the exchange-correlation potential [30] are applied for structure optimizations. The electronic band structure is calculated using hybrid functional proposed by Heyd, Scuseria and Ernzerhof, in which the short-range part of the generalized gradient approximation includes an additional Hartree–Fock contribution [31] . The transition path is simulated with the climbing image nudged elastic band (CI NEB) method [32] . To estimate the threshold energy of irradiation-induced atom displacement, we calculate the non-relaxed formation energy of vacancy as E f = E vac − E perfect + μ x [15] , where E perfect , E vac and μ x are energies of the perfect structure, the non-relaxed structure with mono-vacancy and the removed isolated atom, respectively. For both vacancy’s formation energy and ribbon’s cohesive energy calculation, the spin-polarization was taken into account to determine the chemical potential of an isolated atom. The stress in the tensile simulation was calculated as P = , where d E and d L were the energy and axial constant differences between two loading steps, S was the average cross sectional area with the radius of atoms taken into account. How to cite this article: Liu, X. et al . Top–down fabrication of sub-nanometre semiconducting nanoribbons derived from molybdenum disulphide sheets. Nat. Commun. 4:1776 doi: 10.1038/ncomms2803 (2013). W.G. and L.T.S. conceived the work. X.L. carried out the theoretical investigation. T.X. and X.W. performed the experiments. Z.Z. and J.Y. conducted the energy band calculations. H.Q. and X.R.W. prepared the MoS 2 sample. J.H.H., C.H.J. and J.X.L. conducted the STEM analyses. W.G. organized and wrote the paper with all authors contributed to the discussions and preparation of the manuscript.